A bacterial proteorhodopsin proton pump in marine eukaryotes Proteorhodopsins are light-driven proton pumps involved in widespread phototrophy. Discovered in marine proteobacteria just 10 years ago, proteorhodopsins are now known to have been spread by lateral gene transfer across diverse prokaryotes, but are curiously absent from eukaryotes. In this study, we show that proteorhodopsins have been acquired by horizontal gene transfer from bacteria at least twice independently in dinoflagellate protists. We find that in the marine predator Oxyrrhis marina , proteorhodopsin is indeed the most abundantly expressed nuclear gene and its product localizes to discrete cytoplasmic structures suggestive of the endomembrane system. To date, photosystems I and II have been the only known mechanism for transducing solar energy in eukaryotes; however, it now appears that some abundant zooplankton use this alternative pathway to harness light to power biological functions. A decade ago, a new form of phototrophy based on proteorhodopsin, a novel type of bacterial rhodopsin, was discovered in marine bacterioplankton [1] , [2] . Proteorhodopsin-mediated phototrophy is now known from a wide variety of bacteria and archaea living in diverse environments, and is thought to be spread by horizontal transfer [3] , [4] , [5] . The ecological importance of this process has remained elusive, although evidence shows that it does promote growth and survival in poor conditions [6] , [7] , [8] . In spite of the apparent ease by which these genes spread among prokaryotes, and their subsequent widespread taxonomic distribution, there is as yet no evidence for proteorhodopsin-mediated phototrophy in eukaryotes. Proteorhodopsin is an integral membrane protein that creates a membrane-spanning proton gradient. Unlike bacteria, in which the relatively simple membrane system means that proteorhodopsin can only establish a gradient between the cell and its environment, in eukaryotes the membrane complexity is far greater; therefore, there are numerous compartments in which a gradient can be established, increasing the scope of possible locations and functions for such a system. In this study, we show that one lineage of eukaryotes, dinoflagellates, has acquired multiple types of rhodopsin by horizontal gene transfer from bacteria, including proton-pumping proteorhodopsins of the type used for generating energy from light. In one species previously believed to be strictly heterotrophic, the marine predator Oxyrrhis marina , the protein appears to be functionally significant, as it is the most abundantly expressed nuclear gene and its product localizes to discrete cytoplasmic structures suggestive of the endomembrane system. To date, photosystems I and II have been the only known mechanism for transducing solar energy in eukaryotes; however, it now appears that some abundant zooplankton use this alternative pathway to harness light to power biological functions. Sequence data and phylogenetic analysis We sequenced 18,102 expressed-sequence-tag (EST) from O. marina , which assembled into 9,876 discrete clusters, and found over 40 distinct type-1 rhodopsin genes with a broad range of expression. To address the unlikely possibility that these polyadenylated transcripts are derived from a bacterial contamination and not from O. marina , we examined the 5′ end of the transcripts and found that those not truncated encoded a 5′-spliced leader identical in sequence to the spliced leader found on all dinoflagellate transcripts (including O. marina ), but unknown in any other lineage [9] . This, combined with the finding of a phylogenetically related gene in other dinoflagellates (see below), strongly supports our conclusion that these polyadenylated transcripts are genuine O. marina transcripts and not bacterial contaminants. Phylogenetic analysis ( Fig. 1 ) showed two distantly related families of O. marina rhodopsins. Two distinct but closely related genes encode proteins related to sensory-type rhodopsins [10] from cryptomonad algae, halophilic archaea and fungi (in which a switch to proton-pumping activity may have occurred in at least one species [11] (Dinoflagellate Group 3 in Fig. 1 ). A much larger group of genes was also identified and found to branch within the proton-pumping proteorhodopsins from bacteria (Dinoflagellate Group 1 in Fig. 1 ). Interestingly, ESTs from two other dinoflagellates, Pyrocystis lunula and Alexandrium tamarense , were also identified to branch within this group, as well as a sequence attributed to the marine invertebrate Amphioxus . The Amphioxus sequence is most likely derived from a food or contaminant dinoflagellate, and not from the animal itself, as the sequence is absent from the complete genome. Group 1 dinoflagellate sequences branch with two environmental marine sequences, which in turn form a strongly supported clade with Xanthorhodopsins, a subgroup of proton-pumping proteorhodopsins found in diverse bacteria [12] . A second distinct group of dinoflagellate proteorhodopsins was also identified in Karlodinium micrum (Dinoflagellate Group 2 in Fig. 1 ), which was represented by two closely related genes. Neither of the dinoflagellate proteorhodopsin groups is directly related to any other gene found in a eukaryote; therefore, on the basis of the present distribution they appear to have arisen by horizontal gene transfer from marine bacteria around the origin of dinoflagellates (for Group 1) or within dinoflagellates (for Group 2). 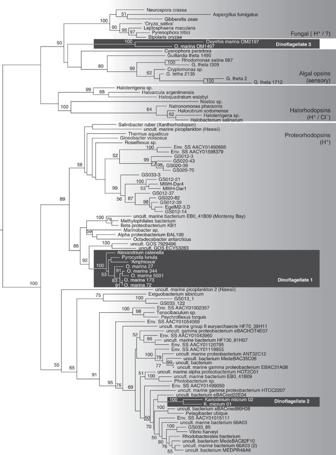Figure 1: Phylogenetic distribution of dinoflagellate rhodopsins. Protein sequences of 96 rhodopsins encompassing the known diversity of microbial (type I) rhodopsins from the three domains of life10were used to generate a maximum likelihood phylogenetic tree (SeeSupplementary Table S1for accession numbers). Grey boxes distinguish the recognized groupings of type 1 rhodopsin, and the prevalent function in each group is shown: proton pumps (H+), sensory, chlorine pumps (Cl−) and unknown (?). Numbers indicate bootstrap support when ≥50% (over 300 replicates). Black boxes highlight dinoflagellate genes: Dinoflagellate 1 is a large group of proteorhodopsins present in diverse dinoflagellates; dinoflagellate 2 includes twoK. micrumproteorhodopsin genes of independent origin; dinoflagellate 3 includes twoO. marinagenes related to algal sensory rhodopsins, probably of endosymbiotic origin. Figure 1: Phylogenetic distribution of dinoflagellate rhodopsins. Protein sequences of 96 rhodopsins encompassing the known diversity of microbial (type I) rhodopsins from the three domains of life [10] were used to generate a maximum likelihood phylogenetic tree (See Supplementary Table S1 for accession numbers). Grey boxes distinguish the recognized groupings of type 1 rhodopsin, and the prevalent function in each group is shown: proton pumps (H + ), sensory, chlorine pumps (Cl − ) and unknown (?). Numbers indicate bootstrap support when ≥50% (over 300 replicates). Black boxes highlight dinoflagellate genes: Dinoflagellate 1 is a large group of proteorhodopsins present in diverse dinoflagellates; dinoflagellate 2 includes two K. micrum proteorhodopsin genes of independent origin; dinoflagellate 3 includes two O. marina genes related to algal sensory rhodopsins, probably of endosymbiotic origin. Full size image Functional properties of dinoflagellate rhodposins Groups 2 and 3 are each restricted to a single species and represented by a small number of ESTs (29 and 12, respectively, from relatively large EST surveys), but Group 1 differs in both respects. On one hand, Group 1 sequences occur in three distantly related dinoflagellates, suggesting an ancient origin in an early ancestor of the lineage. On the other hand, O. marina Group 1 genes are unlike all other eukaryotic rhodopsins in that they form a large gene family, and at least some members of the family are very highly represented in the EST library. Forty distinct genes were identified, and collectively these were represented by 234 ESTs (the most abundant single rhodopsin was represented by 38 ESTs alone), making this the most highly represented nucleus-encoded gene in the survey. Transcripts of many of these genes were confirmed to have the 5′-spliced-leader sequence that is known to be added to all O. marina transcripts [9] . The apparent high level of expression is consistent with the enigmatic bright pink colour of O. marina cells. The same cannot be said for the Group 1 proteorhodopsin from A. tamarensis , represented by a single gene with only four ESTs (there are no data available for the number of ESTs in P. lunula ). The high representation of the O. marina Group 1 rhodopsin is not obviously reconcilable with a sensory role, especially because such a role is more plausibly filled by the O. marina Group 3 genes ( Fig. 1 ). These genes are phylogenetically related to sensory rhodopsins that are involved in phototactic response in cryptophyte algae [13] and in the glaucophyte Cyanophora [14] , where the opsin localizes to the plastid. This scenario suggests that the Group 3 rhodopsins from O. marina were acquired from the ancestral photosynthetic endosymbiont [15] . Alignment with characterized bacterial proteorhodopsin amino-acid sequences and secondary structure prediction of the O. marina protein demonstrate conservation of the seven transmembrane domains and functionally important residues ( Fig. 2a,b ). Notable conserved residues are the proton acceptor Asp in position 101 (97 in eBAC31A08 1 ), the proton donor Glu in position 112 (108 in eBAC31A08 1 ) and the positions predicted to form the retinal pocket including the conserved Lysine (K 237/231 ) that covalently links the retinal [1] , [10] ( Fig. 2a ). Altogether, these features strongly suggest that O. marina proteorhodopsin is a proton pump. Proteorhodopsins in marine bacteria are tuned to maximally absorb the wavelengths of light that predominate at the region of the water column where they tend to occur; green light tuning of proteorhodopsin reflects adaptation to light spectral conditions of surface or near-surface water, whereas blue tuning maximizes attainment of light at deeper levels [2] , [16] , [17] . A specific residue is known to be a useful predictor of this spectral tuning [17] . In the case of O. marina Group 1 rhodopsins, a Leu residue is found at this position 109 (equivalent to position 105 in eBAC31A08 1 : Fig. 2a ), which indicates peak absorption of green light. This is consistent with the ecology of O. marina , which is abundant in tide pools and rocky shores. Interestingly, the dinoflagellate Group 2 sequences from K. micrum have a Glu residue, suggesting tuning to blue light, which may be related to daily vertical migrations, a behaviour exhibited by many dinoflagellates. Altogether, expression levels, phylogenetic origin and sequence characteristics are all consistent with the O. marina Group 1 rhodopsins being an abundant proton-pumping proteorhodopsin derived by horizontal gene transfer from marine bacteria. 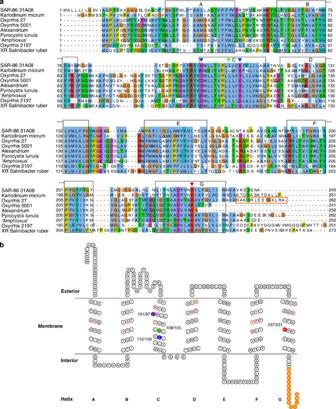Figure 2: Structural and comparative analysis of a dinoflagellate proteorhodopsin. (a) Amino-acid alignment of various rhodopsins from bacteria and dinoflagellates: SAR86-31A08 is a functionally characterized proteorhodopsin1;K. micrumis a 'Dinoflagellate group 2' inFigure 1;Oxyrrhis2197 represents 'Dinoflagellate 3'; XRS. ruberis a Xanthorhodopsin; the remaining sequences belong to 'Dinoflagellate group 1'. Numbers on the right indicate residue number. Black rectangles show predicted transmembrane segments. Functional sites (coloured triangles): blue, proton acceptor and donor; green, spectral tuning (L109/105for green and Q for blue); red, lysine linked to the cofactor retinal. Epitope for antibody preparation is indicated with an orange rectangle. (b) Secondary structure of theO. marinaproteorhodopsin predicted using PHD (http://www.predictprotein.org/). Single-letter amino-acid codes are used, and numbers correspond to the positions inO. marinaand 31A081, respectively. Functional residues are highlighted as follows. Blue: proton acceptor (D101/97) and proton donor (E112/108); green: spectral tuning; red: retinal pocket; red filled: lysine linked to retinal; orange: epitope for antibody. Figure 2: Structural and comparative analysis of a dinoflagellate proteorhodopsin. ( a ) Amino-acid alignment of various rhodopsins from bacteria and dinoflagellates: SAR86-31A08 is a functionally characterized proteorhodopsin [1] ; K. micrum is a 'Dinoflagellate group 2' in Figure 1 ; Oxyrrhis 2197 represents 'Dinoflagellate 3'; XR S. ruber is a Xanthorhodopsin; the remaining sequences belong to 'Dinoflagellate group 1'. Numbers on the right indicate residue number. Black rectangles show predicted transmembrane segments. Functional sites (coloured triangles): blue, proton acceptor and donor; green, spectral tuning (L 109/105 for green and Q for blue); red, lysine linked to the cofactor retinal. Epitope for antibody preparation is indicated with an orange rectangle. ( b ) Secondary structure of the O. marina proteorhodopsin predicted using PHD ( http://www.predictprotein.org/ ). Single-letter amino-acid codes are used, and numbers correspond to the positions in O. marina and 31A08 1 , respectively. Functional residues are highlighted as follows. Blue: proton acceptor (D 101/97 ) and proton donor (E 112/108 ); green: spectral tuning; red: retinal pocket; red filled: lysine linked to retinal; orange: epitope for antibody. Full size image Rhodopsin function requires the prosthetic group retinal, suggesting that retinal biosynthesis should also be present in O. marina . Retinal is one end product of the carotenoid pathway and is formed by splitting β-carotene by a carotenoid dioxygenase. Searching the O. marina ESTs revealed the presence of transcripts encoding a protein with high similarity to carotenoid dioxygenase. We conducted a phylogenetic analysis with diverse carotenoid dioxygenase protein sequences, and the result suggests that O. marina acquired this step of retinal biosynthesis, either horizontally from bacteria or vertically from an ancestral plastid ( Supplementary Fig. S1 ). Unfortunately, the enzyme is not sufficiently well conserved for phylogenetic reconstruction to be more precise. Subcellular localization of rhodopsin in O. marina To determine the subcellular location of the Group 1 proteorhodopsin in O. marina , an antibody was developed against the 14 C-terminal residues shared by several highly expressed copies of the gene ( Fig. 2 ). We tested the antibody specificity by western blotting against total O. marina protein, in which it recognized a single, highly abundant band of the predicted size ( Fig. 3a ). In immunofluorescent subcellular localization, proteorhodopsin was distributed unevenly within the cytosol, indicating some form of cytosolic compartmentalization ( Fig. 3b ). In many but not all cells, a single distinctive ring-like structure was observed ( Fig. 3b , Supplementary Movies 1–4 ). There was no evidence of localization to the plasma membrane, and co-staining with 4,6-diamidino-2-phenylindole and MitoTracker showed no evidence of nuclear or mitochondrial localization of proteorhodopsin ( Fig. 3b ). The ancestor of O. marina possessed a plastid [18] , and relict plastid-targeted protein-coding genes have been found in its nuclear genome [15] ; however, these and other dinoflagellate plastid-targeted proteins encode a distinctive N-terminal-targeting peptide that includes a secretory signal peptide and a distinctive transit peptide [19] . There is no evidence of such a peptide on any O. marina rhodopsin gene, arguing against a location in the hypothetical plastid. Overall, the pattern of proteorhodopsin localization is most consistent with compartmentalization in some fraction of the endomembrane system. We looked for sequences consistent with the characteristics of signal peptides, but the results were inconclusive: some algorithms fail to predict a signal peptide of any sort, whereas others predict a secretory pathway with varying degrees of confidence. If a typical signal peptide is absent, the protein would have to be inserted into the endomembrane from the cytoplasm rather than through the lumen of the endoplasmic reticulum. 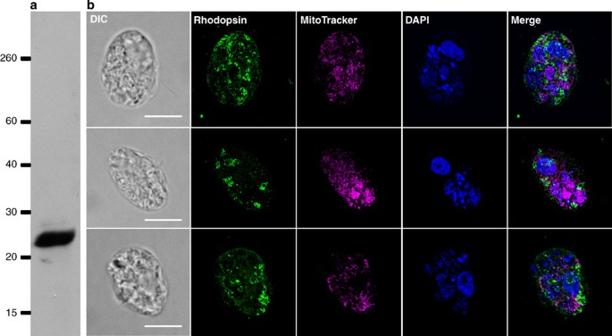Figure 3: Cellular localization of proteorhodopsin inO. marina cells. (a) Western blot of totalO. marinaprotein probed with an antibody raised against the C-terminal peptide of the proteorhodopsin OM27 fromO. marina. Expected protein size is 28 kDa. (b) Localization of proteorhodopsin inO. marinacells using immunofluorescence assay with the same antibody. Antibody signal forms small irregular and ring-like structures independent of mitochondria inO. marina. Three independent cells are shown, each showing (left to right) differential interference contrast (DIC) light micrograph, anti-OM27 proteorhodopsin, MitoTracker staining, Hoechst 33258 staining for DNA and a merge of all four. White bar=10 μm. SeeSupplementary Movies 1–4for a 360° video rendering. DAPI, 4,6-diamidino-2-phenylindole. Figure 3: Cellular localization of proteorhodopsin in O. marina cells . ( a ) Western blot of total O. marina protein probed with an antibody raised against the C-terminal peptide of the proteorhodopsin OM27 from O. marina . Expected protein size is 28 kDa. ( b ) Localization of proteorhodopsin in O. marina cells using immunofluorescence assay with the same antibody. Antibody signal forms small irregular and ring-like structures independent of mitochondria in O. marina . Three independent cells are shown, each showing (left to right) differential interference contrast (DIC) light micrograph, anti-OM27 proteorhodopsin, MitoTracker staining, Hoechst 33258 staining for DNA and a merge of all four. White bar=10 μm. See Supplementary Movies 1–4 for a 360° video rendering. DAPI, 4,6-diamidino-2-phenylindole. Full size image The abundance and diversity of rhodopsins in dinoflagellates is unexpected, given the relatively restricted distribution previously known in eukaryotes, suggesting that rhodopsin perhaps has a variety of sensory or regulatory roles in this lineage. However, the primary structure, localization pattern and expression levels of the Group 1 proteorhodopsin in O. marina all suggest that this protein is a proton pump, highlighting the question of its possible function. Regardless of what this function might be, it must be non-essential in the short term, as it is in prokaryotes, because O. marina can be grown in total darkness. Moreover, the membrane complexity of eukaryotes compounds the number of possibilities significantly, although a couple of more plausible explanations can be singled out. On one hand, the protein might operate very much like its prokaryotic counterparts: if proteorhodopsin is inserted into the same endomembrane compartment as is the vacuolar ATPase (V-ATPase), then its activity would generate a proton gradient that could drive the V-ATPase in reverse, generating energy from light. On the other hand, in a voracious predator such as O. marina , one of the expected functions of V-ATPase is to acidify digestive vacuoles at the expense of ATP; thus, it is also possible that proteorhodopsin replaces or supplements the V-ATPase activity, acidifying digestive vacuoles using light rather than (or besides) ATP. Interestingly, another very highly expressed gene in O. marina is a vacuolar-type H + -pyrophosphatase also found in plants and apicomplexan parasites (a close relative of dinoflagellates). An intriguing possibility is that proteorhodopsin works in conjunction with vacuolar-type H + -pyrophosphatase, generating PPi as an alternative source of energy. In either case, O. marina presents an intriguing mix of feeding strategies that are the sum of a winding path of evolution: the consummate predator that has in the course of evolution shed photosynthesis, only to regain a new version of phototrophy through horizontal gene transfer, perhaps from bacteria on which its ancestors had fed. EST sequencing Oxyrrhis marina strain CCMP1788 was cultivated axenically in Droop's Ox-7 medium. A volume of 20 l of culture was collected in a continuous-flow centrifuge and stored in Trizol (Invitrogen). Total RNA was prepared in 20 ml batches resulting in 2 μg of RNA. A directional cDNA library was constructed in pBluescript II SK using Eco R1 and Xho I sites (Amplicon Express). The library was shown to contain 5.3×10 5 c.f.u., and 23,702 clones were picked and 5′ end-sequenced using Sanger sequencing, and the resulting sequences were assembled using TBestDB ( http://tbestdb.bcm.umontreal.ca ) [20] , yielding 9,876 discrete clusters based on 18,102 ESTs passing quality control. Clusters were compared with public databases using a variety of search strategies and annotated using AutoFACT [21] . Clones corresponding to different types of rhodopsins were identified by sequence similarity with BlastX. Phylogenetic analysis Rhodopsin sequences representing the known subgroups within Type 1 (microbial rhodopsins) were retrieved from GenBank (nr, ests, env) and aligned with Muscle along with a sample of the O. marina rhodopsins. For accession numbers, see Supplementary Table S1 . Sequence management, alignment and manual editing were carried out with the aid of eBiox ( http://www.ebioinformatics.org ). A maximum likelihood phylogenetic tree was constructed using PhyML implemented in Topali [22] . Amino-acid evolution was modelled following the WAG model with four γ-categories and invariable sites. Branch support was assessed with 500 bootstrap replicates. Antibody generation A synthetic peptide with the sequence CNAKSRLEEEGKLRA, identical to the C terminus of the O. marina proteorhodopsin OM27 (see Fig. 3 ), was produced by Genscript and used to immunize two rabbits (as peptide–KLH conjugate). Polyclonal antibodies were affinity-purified and enzyme-linked immunosorbent assay titre was 1:512,000. Western blotting Total cell lysate was extracted using the Mem-PER Eukaryotic Membrane Protein Extraction Kit (Pierce) from a 50 ml culture of O. marina . Proteins were run on 12% SDS–PAGE gels with Neovex Sharp Protein Standards (Invitrogen) and transferred overnight using the mini-PROTEAN gel system (Biorad). Proteorhodopsin was detected using an anti-OM27 O. marina proteorhodopsin antibody (Genscript) with the ONE-HOUR Western Complete Kit (GenScript). Immunofluorescence Preparation was carried out at room temperature unless stated. Cells were collected and incubated in 100 nM MitoTracker Red CMXRos (M7512; Invitrogen) for 30 min, then fixed with 4% formaldehyde and 0.0075% glutaraldehyde in PHEM buffer (60 mM Pipes, 25 mM HEPES, 10 mM EGTA, 2 mM MgCl, pH 7.5) containing 4% NaCl (ref. 23 ) for 30 min on a coverslip coated with 0.01% polyethylenimine. Cells were rinsed once with PHEM buffer, once with PBS, then permeabilized by 0.1% Triton X-100 in PBS for 10 min. Cells were rinsed with PBS and blocked with 0.3% BSA in PBS for 1 h and then incubated with the a-OM27 antibody diluted to 1:10 (initial concentration 0.861 mg ml −1 ) with PBS overnight at 4 °C, rinsed with PBS, then incubated in AlexaFluor-488 goat anti-rabbit IgG (H+L) (A11008; Invitrogen) diluted 1:750 with PBS for 1 h, rinsed with PBS, incubated with Hoechst 33258 (H1398; Invitrogen) for 10 min, rinsed and finally mounted with 1% 1,4-diazabicyclo[2,2,2]octane (D-2522; Sigma-Aldrich) in 90% glycerol. Cells were observed using a Perkin Elmer UltraView VoX Spinning Disk Confocal microscope consisting of a Leica DMI6000 inverted microscope equipped with a customized Hamamatsu 9100-02. Images were obtained and deconvoluted with Volocity ver.5 software (Improvision), and then post-processed on ImageJ ver.1.43u (ref. 24 ). Accession codes: New nucleotide sequences have been deposited in GenBank under accession numbers HQ654763 to HQ654769 . How to cite this article: Slamovits, C. H. et al . A bacterial proteorhodopsin proton pump in marine eukaryotes. Nat. Commun. 2:183 doi: 10.1038/ncomms1188 (2011).